Mechanistic insight into GPCR-mediated activation of the microtubule-associated RhoA exchange factor GEF-H1 The RhoGEF GEF-H1 can be sequestered in an inactive state on polymerized microtubules by the dynein motor light-chain Tctex-1. Phosphorylation of GEF-H1 Ser885 by PKA or PAK kinases creates an inhibitory 14-3-3-binding site. Here we show a new mode of GEF-H1 activation in response to the G-protein-coupled receptor (GPCR) ligands lysophosphatidic acid (LPA) or thrombin that is independent of microtubule depolymerization. LPA/thrombin stimulates disassembly of the GEF-H1:dynein multi-protein complex through the concerted action of Gα and Gβγ. Gα binds directly to GEF-H1 and displaces it from Tctex-1, while Gβγ binds to Tctex-1 and disrupts its interaction with the dynein intermediate chain, resulting in the release of GEF-H1. Full activation of GEF-H1 requires dephosphorylation of Ser885 by PP2A, which is induced by thrombin. The coordinated displacement of GEF-H1 from microtubules by G-proteins and its dephosphorylation by PP2A demonstrate a multistep GEF-H1 activation and present a unique mechanism coupling GPCR signalling to Rho activation. The Rho GTPases are critical modulators of cell morphology and motility through their regulation of the actin cytoskeleton. The activation state of Rho GTPases is governed by the balance between the activities of GTPase-activating proteins, which catalyse hydrolysis of guanosine-5′-triphosphate (GTP) and guanine exchange factors (GEFs), which promote GTP binding. GEF-H1, also known as ARHGEF2 or Lfc in mouse, is associated with microtubules in its inactive state [1] . Expression of GEF-H1 promotes stress fibre formation through RhoA activation, while its depletion attenuates actin reorganization [2] , [3] , [4] , [5] . A mutant of GEF-H1 unable to bind to microtubules has increased GEF activity and induces stress fibre formation [5] , suggesting that GEF-H1 is a critical factor mediating crosstalk between microtubules and actin [5] . We have shown that the dynein light-chain Tctex-1 tethers GEF-H1 to polymerized microtubules [6] , where it is poised to undergo D-AKAP-1-dependent phosphorylation of Ser885 by PKA. Phosphorylation of Ser885 creates a high-affinity 14-3-3-binding site that inhibits the exchange activity of GEF-H1 (ref. 3 ). Nocodazole-induced depolymerization of microtubules disrupts this inhibited GEF-H1 complex resulting in potent activation of GEF-H1, suggesting that cycles of microtubule depolymerization under physiologic conditions would release GEF-H1, providing local and temporally constrained activation of RhoA [6] , [7] . We and others have shown that a variety of receptor ligands including lysophosphatidic acid (LPA) [3] , thrombin [2] , tumour necrosis factor-α and epidermal growth factor [8] , [9] lead to activation of GEF-H1 through unknown mechanisms. Moreover, GEF-H1 can be activated by mechanotransduction through an integrin-mediated mechanism, which is suggested to be independent of microtubule depolymerization [10] . In the present study, we sought to determine the mechanism underlying GEF-H1 activation in response to the GPCR (G-protein-coupled receptor) ligands LPA and thrombin. Gα 12/13 proteins play a well-established role in the activation of RhoGEFs belonging to the regulator of G-protein signalling (RGS) domain-containing RhoGEF subfamily, which includes p115-RhoGEF, PDZ-RhoGEF, leukemia-associated RhoGEF (LARG) and possibly Lbc-RhoGEF [11] , [12] , [13] . Gα 12/13 subunits bind directly to the RGS-homology (RH) domain contained within the polypeptide sequences of these GEFs, which is thought to alleviate autoinhibition of their exchange activity. Although GEF-H1 is known to respond to Gα 12/13 -coupled GPCR stimulation, to date no interaction with Gα 12/13 has been shown, nor has an RH domain been identified in its polypeptide sequence. Here we identify a novel mechanism for GEF-H1 activation mediated by the coincident interaction of Gα 12/13 with GEF-H1 and Gβγ with Tctex-1, resulting in the release and activation of GEF-H1 from the inhibitory dynein-associated complex. In addition, we show that thrombin stimulates the interaction between PP2A and GEF-H1 triggering dephosphorylation of Ser885, which is required for activation. This study provides a detailed multistep mechanism for GPCR-mediated activation of GEF-H1 independent of microtubule depolymerization. LPA/thrombin induce GEF-H1 release from intact microtubules GEF-H1 is required for LPA/thrombin-induced stress fibre formation, and focal adhesion formation following stimulation with tumour necrosis factor-α, LPA or thrombin [2] , [3] , [6] . We have recently shown that microtubule-dependent inhibition of GEF-H1 requires the assembly of a protein complex including Tctex-1, dynein intermediate chain (DIC) and 14-3-3 proteins [6] . We examined whether the microtubule-associated inhibited GEF-H1 complex is altered following LPA or thrombin stimulation, and observed that 5 min following treatment with LPA or thrombin, the stoichiometry of DIC, 14-3-3 and Tctex-1 present in GEF-H1 immune complexes markedly decreased compared with basal conditions ( Fig. 1a ). 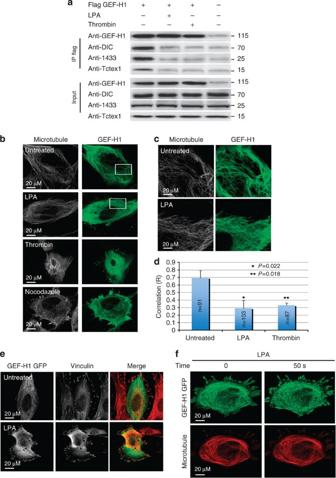Figure 1: GEF-H1 translocates from microtubules to the cytoplasm and focal adhesions in response to LPA or thrombin. (a) LPA or thrombin treatment disrupts GEF-H1–dynein complex. Serum-starved HEK293T cells, expressing Flag-tagged GEF-H1, were treated with LPA or thrombin for 5 min. Endogenous DIC, 14-3-3 and Tctex-1 proteins were detected in Flag-GEF-H1-precipitated complexes by western blot. Western blots of the whole-cell lysate (input) and immunoprecipitated complexes (IP) are shown. (b) LPA or thrombin induced GEF-H1 relocalization from microtubules. Confocal images of GEF-H1−/−MEFs transfected with GEF-H1–eGFP were treated with LPA, thrombin or nocodazole, as indicated, for 5 min prior to fixation and staining with anti-tubulin. Scale bar, 20 μm. (c) Higher magnification (5 × 60) view of the images depicted inb. Scale bar, 20 μm. (d) The correlation coefficient (R) measuring co-localization between eGFP (GEF-H1) and polymerized microtubules inbwas determined in 90 cells from three independent experiments. Error bars represent s.d. of at least three independent replicates, andPvalues derived from pairwiset-tests are indicated. (e) GEF-H1 translocates to focal adhesions in response to LPA. GEF-H1−/−MEFs overexpressing GEF-H1–eGFP were treated with LPA for 1 h prior to fixation and staining with anti-vinculin antibodies (red) to visualize focal adhesions. Co-localization between GEF-H1 (GFP) and vinculin was measured with and without LPA treatment. Scale bar, 20 μm. (f) GEF-H1 relocalization using live-cell imaging. Images from movies of GEF-H1−/−MEF cells transiently transfected with GEF-H1–eGFP and cherry tubulin, before and after LPA stimulation. Starved cells were treated with LPA. Data are representative of three independent biological replicates. Scale bar, 20 μm. Figure 1: GEF-H1 translocates from microtubules to the cytoplasm and focal adhesions in response to LPA or thrombin. ( a ) LPA or thrombin treatment disrupts GEF-H1–dynein complex. Serum-starved HEK293T cells, expressing Flag-tagged GEF-H1, were treated with LPA or thrombin for 5 min. Endogenous DIC, 14-3-3 and Tctex-1 proteins were detected in Flag-GEF-H1-precipitated complexes by western blot. Western blots of the whole-cell lysate (input) and immunoprecipitated complexes (IP) are shown. ( b ) LPA or thrombin induced GEF-H1 relocalization from microtubules. Confocal images of GEF-H1 −/− MEFs transfected with GEF-H1–eGFP were treated with LPA, thrombin or nocodazole, as indicated, for 5 min prior to fixation and staining with anti-tubulin. Scale bar, 20 μm. ( c ) Higher magnification (5 × 60) view of the images depicted in b . Scale bar, 20 μm. ( d ) The correlation coefficient ( R ) measuring co-localization between eGFP (GEF-H1) and polymerized microtubules in b was determined in 90 cells from three independent experiments. Error bars represent s.d. of at least three independent replicates, and P values derived from pairwise t -tests are indicated. ( e ) GEF-H1 translocates to focal adhesions in response to LPA. GEF-H1 −/− MEFs overexpressing GEF-H1–eGFP were treated with LPA for 1 h prior to fixation and staining with anti-vinculin antibodies (red) to visualize focal adhesions. Co-localization between GEF-H1 (GFP) and vinculin was measured with and without LPA treatment. Scale bar, 20 μm. ( f ) GEF-H1 relocalization using live-cell imaging. Images from movies of GEF-H1 −/− MEF cells transiently transfected with GEF-H1–eGFP and cherry tubulin, before and after LPA stimulation. Starved cells were treated with LPA. Data are representative of three independent biological replicates. Scale bar, 20 μm. Full size image Dissolution of the interaction between DIC–Tctex-1 and GEF-H1 might represent one mechanism by which growth factor stimulation could activate GEF-H1 by displacement from the microtubule array. We investigated whether LPA or thrombin stimulation alters GEF-H1 localization. GEF-H1-knockout murine embryonic fibroblasts (MEFs) were transfected with GEF-H1–enhanced green fluorescent protein (eGFP) and visualized by confocal microscopy before and after treatment. In untreated cells, GEF-H1–eGFP was closely associated with the microtubule array (correlation coefficient of 0.67, n =91), whereas after 5 min of LPA or thrombin treatment GEF-H1–eGFP moved into a largely cytoplasmic distribution ( Fig. 1b–d ). Similar to GEF-H1 localization after application of force [10] , we noted that a fraction of GEF-H1 relocalized to vinculin-positive focal adhesion structures following treatment with LPA (correlation coefficient of 0.81, n =74) ( Fig. 1e ; Supplementary Fig. 1 ). Importantly, acute treatment with LPA or thrombin did not depolymerize the microtubule network, suggesting that under these conditions GEF-H1 displacement was not contingent on disruption of microtubule arrays ( Fig. 1c ). To address the possibility that growth factor stimulation of cells increased microtubule dynamics, which may not be observable under steady-state conditions, we visualized live cells expressing cherry tubulin and GEF-H1–eGFP using real-time confocal microscopy. Live imaging verified that the bulk of the microtubule array remained intact during the time interval of the stimulation coincident with GEF-H1 relocalization into the cytoplasm ( Fig. 1f ). The Gβ subunit binds to Tctex-1 and activates GEF-H1 LPA and thrombin signal to cells through activation of the LPA receptors and protease-activated GPCRs, respectively. Inactive GPCRs associate with α-, β- and γ-subunits (known as Gα, Gβ and Gγ, respectively), however, upon ligand activation, the Gα subunit dissociates from the Gβγ heterodimer, where upon both subunits can engage multiple intracellular signalling pathways. Sachdev et al . [15] showed that the Gβ subunit binds to Tctex-1 and competes with DIC for binding to Tctex-1, regulating assembly of Tctex-1 into the dynein motor complex [14] , [15] . We asked whether Gβγ subunits might impinge on the GEF-H1:Tctex-1:dynein complex, leading to the displacement of GEF-H1 from microtubules and its activation. We confirmed that Gβ bound to Tctex-1 in 293T cells co-expressing Gβ 12 isoform, Tctex-1 and GEF-H1, while a Gβ variant (Gβ mut ) bearing three mutations (R48A, R49A and R52A) in the Tctex-1-binding site pulled down significantly less Tctex-1 ( Fig. 2a ), consistent with results reported by Sachdev et al . [15] To determine whether Gβ binding to Tctex-1 disrupts the interaction between GEF-H1 and Tctex-1, GEF-H1 immune complexes were analysed for the presence of Tctex-1 in the absence or presence of the expressed Gβ 12 subunit. While Tctex-1 was detected in GEF-H1 immunoprecipitates, expression of Gβ markedly reduced the association of GEF-H1 with Tctex-1 protein ( Fig. 2b ). The specificity of this effect was demonstrated by the observation that Gβ mut expression did not alter the GEF-H1:Tctex-1 interaction ( Fig. 2b ). These data suggest that the Gβ subunit can disrupt the anchoring function of Tctex-1 that links GEF-H1 to microtubules. We therefore examined whether Gβ 12 γ 12 expression could alter GEF-H1 localization to the microtubule array using fluorescence microscopy. We observed that the localization of GEF-H1–eGFP, normally intimately associated with the microtubule array, redistributed into a diffuse pattern in cells expressing the Gβγ subunits ( Fig. 2c ; Supplementary Fig. 2a ). To demonstrate the specificity of the Gβγ effect on GEF-H1 redistribution, we co-expressed the Gβγ-specific antagonist peptide, βARKct, derived from the Gβγ-binding domain of β-adrenergic receptor kinase 1, which specifically inhibits Gβγ-dependent signalling [16] , and noted that co-expression of βARKct restored GEF-H1–eGFP localization to the microtubules ( Fig. 2c ; Supplementary Fig. 2a ). We next queried whether Gβγ expression could induce stress fibre formation in a GEF-H1-dependent manner following the redistribution of GEF-H1 from the microtubule array. We found that expression of the Gβγ subunits was sufficient to induce actin-based stress fibres in wild-type MEFs but not in GEF-H1 knockout MEFs ( Fig. 2d ), reinforcing the idea that Gβγ plays a role in inducing stress fibre formation through GEF-H1. Last, we investigated whether expression of Gβγ could regulate the catalytic activity of GEF-H1. As previously reported, Tctex-1 potently inhibited the exchange activity of full-length GEF-H1 (refs 6 , 17 ), whereas co-expression of the Gβγ subunits relieved this inhibitory effect ( Fig. 2e ). In contrast, expression of the Gβ mut peptide was unable to antagonize the inhibitory effect of Tctex-1 ( Fig. 2e ; Supplementary Fig. 2b ). Co-expression of the βARKct inhibitory peptide blocked the ability of Gβγ to antagonize Tctex-1-mediated inhibition of GEF-H1 ( Fig. 2e ; Supplementary Fig. 2b ), demonstrating the specificity of the Gβγ effect. These data demonstrate that Gβγ can disrupt the interaction of GEF-H1 with the dynein motor complex leading to its displacement from the microtubule array and activation of its exchange activity. 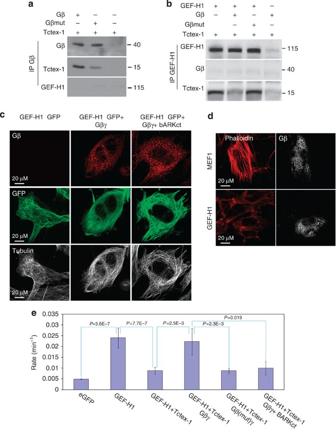Figure 2: Gβ subunit binds to Tctex-1 and activates GEF-H1. (a) Gβ subunit binds Tctex-1 in HEK293T cells. Flag-Tctex-1 was expressed in HEK293T cells alone or co-expressed with Gβ or a Gβ variant with mutations at the Tctex-1-binding site (Gβmut,R48A, R49A and R52A). Cells were lysed and Gβ protein complexes precipitated with anti-Gβ antibody were probed with anti-Gβ, anti-Tctex-1 and anti-GEF-H1 antibodies. (b) Gβ displaces GEF-H1 from Tctex-1. Myc-GEF-H1 and Flag-Tctex-1 were expressed with Gβ12or Gβmutin HEK293T cells, and following lysis, GEF-H1 complexes were immunoprecipitated with anti-Myc antibody, and probed with anti-Gβ, anti-Tctex-1 or anti-GEF-H1 antibodies, respectively. (c) Gβ12γ12overexpresion induces GEF-H1 relocalization. Confocal images of GEF-H1−/−cells expressing GEF-H1–eGFP or co-expressing GEF-H1–eGFP and Gβ12γ12, with or without βARKct (Gβγ-specific antagonist). Cells were fixed 1 day after transfection and stained with anti-Gβ or α-tubulin antibodies. Scale bar, 20 μm. (d) Gβ12γ12expression induces stress fibre formation in a GEF-H1-dependent manner. Wild-type or GEF-H1−/−MEFs, expressing Gβ12γ12proteins, were fixed 1 day after transfection, stained with anti-Gβ and anti-phalloidin antibodies and visualized by confocal microscopy. Scale bar, 20 μm. (e) Gβγ expression activates GEF-H1 exchange activity in a specific manner. RhoA nucleotide exchange rates in the presence of lysates derived from HEK293T cells overexpressing eGFP alone, GEF-H1–eGFP or co-expressing GEF-H1–eGFP and Flag-Tctex-1 with or without co-transfection of Gβγ, Gβmutγ or Gβγ and the inhibitory βARKct peptide. GEF-H1, Tctex-1 and Gβ protein levels in cell lysates were detected by western blots. Error bars represent s.d. of at least three independent replicates, andPvalues derived from pairwiset-tests are indicated. Figure 2: Gβ subunit binds to Tctex-1 and activates GEF-H1. ( a ) Gβ subunit binds Tctex-1 in HEK293T cells. Flag-Tctex-1 was expressed in HEK293T cells alone or co-expressed with Gβ or a Gβ variant with mutations at the Tctex-1-binding site (Gβ mut, R48A, R49A and R52A). Cells were lysed and Gβ protein complexes precipitated with anti-Gβ antibody were probed with anti-Gβ, anti-Tctex-1 and anti-GEF-H1 antibodies. ( b ) Gβ displaces GEF-H1 from Tctex-1. Myc-GEF-H1 and Flag-Tctex-1 were expressed with Gβ 12 or Gβ mut in HEK293T cells, and following lysis, GEF-H1 complexes were immunoprecipitated with anti-Myc antibody, and probed with anti-Gβ, anti-Tctex-1 or anti-GEF-H1 antibodies, respectively. ( c ) Gβ 12 γ 12 overexpresion induces GEF-H1 relocalization. Confocal images of GEF-H1 −/− cells expressing GEF-H1–eGFP or co-expressing GEF-H1–eGFP and Gβ 12 γ 12 , with or without βARKct (Gβγ-specific antagonist). Cells were fixed 1 day after transfection and stained with anti-Gβ or α-tubulin antibodies. Scale bar, 20 μm. ( d ) Gβ 12 γ 12 expression induces stress fibre formation in a GEF-H1-dependent manner. Wild-type or GEF-H1 −/− MEFs, expressing Gβ 12 γ 12 proteins, were fixed 1 day after transfection, stained with anti-Gβ and anti-phalloidin antibodies and visualized by confocal microscopy. Scale bar, 20 μm. ( e ) Gβγ expression activates GEF-H1 exchange activity in a specific manner. RhoA nucleotide exchange rates in the presence of lysates derived from HEK293T cells overexpressing eGFP alone, GEF-H1–eGFP or co-expressing GEF-H1–eGFP and Flag-Tctex-1 with or without co-transfection of Gβγ, Gβ mut γ or Gβγ and the inhibitory βARKct peptide. GEF-H1, Tctex-1 and Gβ protein levels in cell lysates were detected by western blots. Error bars represent s.d. of at least three independent replicates, and P values derived from pairwise t -tests are indicated. Full size image Gα 12/13 subunit induces GEF-H1 localization and activation Gα 12/13 subunits directly activate a class of RhoGEFs including p115-RhoGEF, PDZ-RhoGEF, LARG and Lbc-RhoGEF [11] , [12] that contain Gα-binding RH domains. LPA or thrombin signalling through Gα 12/13 subunits induces stress fibres in a manner that requires GEF-H1 (ref. 5 ), yet GEF-H1 does not have an identifiable RGS domain. We directly tested whether the induction of stress fibres by Gα 12 and Gα 13 was dependent on GEF-H1. We observed that wild-type, but not GEF-H1-knockout, MEFs expressing Gα 12 or Gα 13 subunits contained high levels of polymerized actin ( Fig. 3a ; Supplementary Fig. 3 ). The requirement of GEF-H1 for stress fibre formation suggested that this aspect of Gα 12/13 signalling operates through the GEF-H1 pathway. We next examined whether constitutively active Gα 12 or Gα 13 could trigger a change in GEF-H1 localization and stimulate GEF-H1 activation. GEF-H1 −/− cells were transfected with GEF-H1–eGFP alone or together with a constitutively active Gα 12/13 mutant (Gα 12QL, Gα 13QL ), fixed and stained with phalloidin or anti-tubulin antibodies. GEF-H1–eGFP localized to microtubules in starved cells that contained little polymerized actin ( Fig. 3b,c ; Supplementary Fig. 3 ). Expression of Gα 12QL or Gα 13QL induced the redistribution of GEF-H1–eGFP from the microtubule array to a diffuse cytoplasmic pattern and was associated with stress fibre formation ( Fig. 3b,c ; Supplementary Fig. 3 ), both of which were blocked by the co-expression of the RGS domain of p115 (rgRGS), which specifically binds and blocks Gα 12/13 (refs 18 , 19 ). This demonstrates that the RH domain-binding surface of Gα 12QL is required to regulate GEF-H1 redistribution from the microtubules. 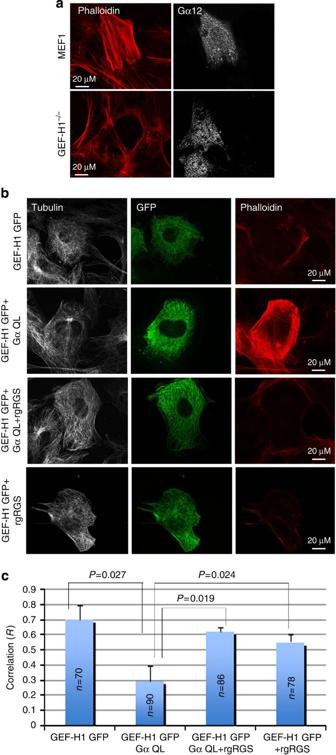Figure 3: Gα12induces translocation and activation of GEF-H1. (a) Induction of stress fibres by Gα12requires GEF-H1. Wild-type or GEF-H1−/−MEFs ectopically expressing Gα12were stained with anti-phalloidin or anti-Gα12antibodies and imaged by confocal microscopy. Scale bar, 20 μm. (b) Gα12expression triggers GEF-H1 relocalization and activation. GEF-H1−/−cells were transfected with GEF-H1–eGFP alone or together with a constitutively active Gα12(GαQL) mutant or with GαQLand dominant-negative RGS peptide (rgRGS). Cells were stained with anti-phalloidin or anti-tubulin antibodies and imaged. Scale bar, 20 μm. (c) The correlation coefficient of GEF-H1–eGFP and polymerized microtubules co-localization inbwas determined in 70 cells (or more) from three independent experiments. Error bars represent s.d. of at least three independent replicates, andPvalues derived from pairwiset-tests are indicated. Figure 3: Gα 12 induces translocation and activation of GEF-H1. ( a ) Induction of stress fibres by Gα 12 requires GEF-H1. Wild-type or GEF-H1 −/− MEFs ectopically expressing Gα 12 were stained with anti-phalloidin or anti-Gα 12 antibodies and imaged by confocal microscopy. Scale bar, 20 μm. ( b ) Gα 12 expression triggers GEF-H1 relocalization and activation. GEF-H1 −/− cells were transfected with GEF-H1–eGFP alone or together with a constitutively active Gα 12 (Gα QL ) mutant or with Gα QL and dominant-negative RGS peptide (rgRGS). Cells were stained with anti-phalloidin or anti-tubulin antibodies and imaged. Scale bar, 20 μm. ( c ) The correlation coefficient of GEF-H1–eGFP and polymerized microtubules co-localization in b was determined in 70 cells (or more) from three independent experiments. Error bars represent s.d. of at least three independent replicates, and P values derived from pairwise t -tests are indicated. Full size image The Gα subunit binds directly to GEF-H1 To determine whether activation of GEF-H1 by Gα 12/13 is mediated by a direct binding event, we performed pull-down experiments with purified recombinant Gα 13 (a chimera of Gα i1 residues 1–28 fused to Gα 13 residues 41–377 (ref. 20 )) and GEF-H1 proteins. Recombinant full-length GEF-H1 protein expressed and purified from insect cells [6] bound to recombinant Gα 13 , indicating that active Gα can bind directly to GEF-H1 in vitro ( Supplementary Fig. 4a ). A series of GEF-H1 truncations and deletions revealed that the Gα 12/13 -binding site resides in the N-terminal region of GEF-H1 ( Fig. 4a ; Supplementary Fig. 4b ). Co-immunoprecipitation experiments with a series of Flag-tagged, N-terminal expressed GEF-H1 fragments demonstrated that amino acids 1–240 of GEF-H1 are sufficient for optimal binding to endogenous Gα 12 while shorter deletions within this region markedly reduced Gα binding ( Fig. 4b ). The requirement for the entire 240-a.a. N terminus of GEF-H1 for Gα binding suggests either the presence of a folded domain or several multivalent-binding sites, and is consistent with the size of RH domains of p115, PDZ and LARG, which are 200 amino acids or greater in length. 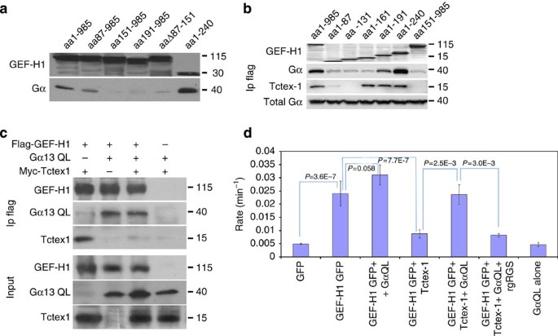Figure 4: The Gα12/13subunit binds to GEF-H1, displaces Tctex-1 and stimulates exchange activity. (a) The Gα-binding site resides in theN-terminal region of GEF-H1. His-GEF-H1 (a.a. 1–985) or a series of N- and C-terminal truncations and deletions were expressed in HEK293T cells and protein complexes were immunoprecipitated with α-His antibodies. GEF-H1 immune complexes were immunoblotted with anti-GEF-H1 or anti-Gα13antibodies. (b) Optimal binding to endogenous Gα13requires the first 240 amino acids of GEF-H1. Flag-GEF-H1 or a series ofN-terminal fragments were expressed in HEK293T cells and protein complexes were immunoprecipitated with anti-Flag antibodies. GEF-H1 immune complexes were immunoblotted with anti-GEF-H1, anti-Gα13or anti-Tctex-1 antibodies to detect endogenous Gα13and Tctex-1, respectively. Total Gα13levels were assessed by western blot. (c) Constitutively active Gα13inhibits the association of Tctex-1 with GEF-H1. Flag complexes were immunoprecipitated from HEK293T lysates expressing Flag-GEF-H1 with or without Myc-Tctex-1 and Gα13QL, and immunoblotted with anti-GEF-H1, anti-Tctex-1 or anti-Gα13antibodies. Western blot of GEF-H1, Gα13and Tctex-1 are shown. (d) Gα13QLantagonizes Tctex-1-mediated inhibition of GEF-H1 exchange activity. RhoA nucleotide exchange rates were measured in lysates from HEK293T cells expressing combinations of eGFP, GEF-H1–eGFP, Flag-Tctex-1, constitutively active Gα13QLand the inhibitory rgRGS domain, as indicated. GEF-H1, Tctex-1 and GαQLexpression were confirmed by western blots. The s.d. derived from at least three independent replicate experiments are shown along withPvalues from pairwiset-tests. Figure 4: The Gα 12/13 subunit binds to GEF-H1, displaces Tctex-1 and stimulates exchange activity. ( a ) The Gα-binding site resides in the N -terminal region of GEF-H1. His-GEF-H1 (a.a. 1–985) or a series of N- and C-terminal truncations and deletions were expressed in HEK293T cells and protein complexes were immunoprecipitated with α-His antibodies. GEF-H1 immune complexes were immunoblotted with anti-GEF-H1 or anti-Gα 13 antibodies. ( b ) Optimal binding to endogenous Gα 13 requires the first 240 amino acids of GEF-H1. Flag-GEF-H1 or a series of N -terminal fragments were expressed in HEK293T cells and protein complexes were immunoprecipitated with anti-Flag antibodies. GEF-H1 immune complexes were immunoblotted with anti-GEF-H1, anti-Gα 13 or anti-Tctex-1 antibodies to detect endogenous Gα 13 and Tctex-1, respectively. Total Gα 13 levels were assessed by western blot. ( c ) Constitutively active Gα 13 inhibits the association of Tctex-1 with GEF-H1. Flag complexes were immunoprecipitated from HEK293T lysates expressing Flag-GEF-H1 with or without Myc-Tctex-1 and Gα 13QL , and immunoblotted with anti-GEF-H1, anti-Tctex-1 or anti-Gα 13 antibodies. Western blot of GEF-H1, Gα 13 and Tctex-1 are shown. ( d ) Gα 13QL antagonizes Tctex-1-mediated inhibition of GEF-H1 exchange activity. RhoA nucleotide exchange rates were measured in lysates from HEK293T cells expressing combinations of eGFP, GEF-H1–eGFP, Flag-Tctex-1, constitutively active Gα 13QL and the inhibitory rgRGS domain, as indicated. GEF-H1, Tctex-1 and Gα QL expression were confirmed by western blots. The s.d. derived from at least three independent replicate experiments are shown along with P values from pairwise t -tests. Full size image The Gα-binding site on GEF-H1 overlaps the binding site of Tctex-1. Therefore, we asked whether Gα 12/13 competes with Tctex-1 binding, and whether displacement of Tctex-1 by Gα 12/13 may contribute to the activation of GEF-H1. GEF-H1 immune complexes from HEK293T cells expressing GEF-H1, Tctex-1 and Gα 13QL were analysed for the presence of Tctex-1 and Gα 13 . While Tctex-1 was detected in GEF-H1 immunoprecipitates derived from cells expressing GEF-H1 and Tctex-1 alone, expression of Gα 13QL markedly reduced the association of Tctex-1 with GEF-H1 ( Fig. 4c ). Moreover, Gα 13QL potently antagonized the inhibition of GEF-H1 exchange activity by overexpressed Tctex-1 in an rgRGS-sensitive manner ( Fig. 4d ), consistent with the observation that Gα 13QL functionally competes with Tctex-1. In the absence of Tctex-1 overexpression, GEF-H1 exchange activity increased when Gα 13QL was co-expressed, however, this trend did not reach statistical significance, supporting the hypothesis that displacement of Tctex-1 is the major mechanism by which Gα 13 activates GEF-H1. Similar results were obtained for Gα 12QL . We and others have previously shown that GEF-H1 is phosphorylated on Ser885 and associated with 14-3-3 proteins in its inactive state [3] , [21] . We examined whether Gα 13QL disrupted the interaction of 14-3-3 with GEF-H1 as a surrogate measure of GEF-H1 activation. We probed the association of 14-3-3 with GEF-H1 in cells with or without Gα 13QL expression. While 14-3-3 was detected in GEF-H1 immunoprecipitates derived from GEF-H1-transfected cells, Gα 13QL co-expression markedly reduced the association of 14-3-3 proteins with GEF-H1 ( Fig. 5a ). Expression of the dominant-negative rgRGS domain blocked this effect of Gα 13QL , and restored the interaction between 14-3-3 and GEF-H1 ( Fig. 5a ). We next co-expressed GEF-H1 with 14-3-3 or Tctex-1 or Gα 13QL , immunoprecipitated 14-3-3, Tctex-1 or Gα 13QL and probed the status of Ser885 phosphorylation in each complex with a phospho-Ser885-specific GEF-H1 antibody. We observed that the level of GEF-H1 Ser885 phosphorylation was strongly correlated with association with 14-3-3 and Tctex-1 and inversely correlated with Gα 13 association ( Fig. 5b ). These results suggest that GEF-H1 bound to Gα is in its active state (that is, dephosphorylated on Ser885). 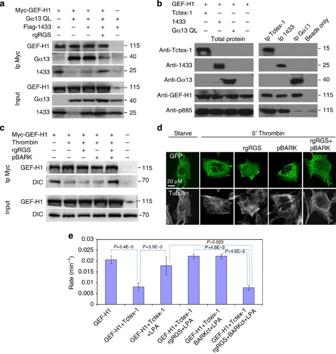Figure 5: Gα12/13signalling reduces the interaction of 14-3-3 with GEF-H1 and can stimulate exchange activity independent of Gβ. (a) Gα13QLdisrupts 14-3-3 protein interaction with GEF-H1. HEK293T cells were transfected with Myc-GEF-H1 with or without Flag-14-3-3 and Gα13QL, or with the dominant-negative RGS peptide (rgRGS). Myc-protein complexes were immunoblotted with anti-GEF-H1, anti-Flag or anti-Gα13antibodies. Western blots of GEF-H1, Gα13and 14-3-3 in the whole-cell lysate are shown. (b) Gα13-bound GEF-H1 is dephosphorylated at Ser885. HEK293T cells were transfected with GEF-H1, Flag-Tctex-1, Myc-14-3-3 and Gα13QL. Myc- Flag- and Gα13protein complexes were precipitated from lysates and immunoblotted with anti-Tctex-1, anti-14-3-3, anti-Gα13, anti-GEF-H1 or anti-phosphoSer885 antibodies (right panel). Western blots of total cell lysates are shown (left). (c) Inhibition of both Gα and Gβ are required to inhibit thrombin-induced disruption of the GEF-H1–dynein complex. Cells were transfected with Myc-GEF-H1 with or without rgRGS and/or βARKct. Cells were treated with thrombin and Myc-complexes were immunoprecipitated from lysates and blotted for endogenous GEF-H1 and DIC. Western blots of total GEF-H1 and DIC are shown below. (d) Inhibition of both Gα and Gβ are required to block thrombin-induced relocalization of GEF-H1. GEF-H1−/−cells were transfected with GEF-H1–eGFP alone or with rgRGS and/or βARKct. Cells were treated with thrombin, fixed and stained with anti-α-tubulin antibodies and imaged by confocal microscopy. Scale bar, 20 μm. (e) Inhibition of both Gα and Gβ are required to block LPA-induced activation of GEF-H1 exchange activity. RhoA nucleotide exchange rates were measured in lysates from HEK293T cells expressing combinations of GEF-H1–eGFP, Tctex-1, rgRGS domain and βARKct peptide, with or without LPA stimulation, as indicated. The s.d. of at least three independent replicates are shown along withPvalues from pairwiset-tests. Figure 5: Gα 12/13 signalling reduces the interaction of 14-3-3 with GEF-H1 and can stimulate exchange activity independent of Gβ. ( a ) Gα 13QL disrupts 14-3-3 protein interaction with GEF-H1. HEK293T cells were transfected with Myc-GEF-H1 with or without Flag-14-3-3 and Gα 13QL , or with the dominant-negative RGS peptide (rgRGS). Myc-protein complexes were immunoblotted with anti-GEF-H1, anti-Flag or anti-Gα 13 antibodies. Western blots of GEF-H1, Gα 13 and 14-3-3 in the whole-cell lysate are shown. ( b ) Gα 13 -bound GEF-H1 is dephosphorylated at Ser885. HEK293T cells were transfected with GEF-H1, Flag-Tctex-1, Myc-14-3-3 and Gα 13QL . Myc- Flag- and Gα 13 protein complexes were precipitated from lysates and immunoblotted with anti-Tctex-1, anti-14-3-3, anti-Gα 13 , anti-GEF-H1 or anti-phosphoSer885 antibodies (right panel). Western blots of total cell lysates are shown (left). ( c ) Inhibition of both Gα and Gβ are required to inhibit thrombin-induced disruption of the GEF-H1–dynein complex. Cells were transfected with Myc-GEF-H1 with or without rgRGS and/or βARKct. Cells were treated with thrombin and Myc-complexes were immunoprecipitated from lysates and blotted for endogenous GEF-H1 and DIC. Western blots of total GEF-H1 and DIC are shown below. ( d ) Inhibition of both Gα and Gβ are required to block thrombin-induced relocalization of GEF-H1. GEF-H1 −/− cells were transfected with GEF-H1–eGFP alone or with rgRGS and/or βARKct. Cells were treated with thrombin, fixed and stained with anti-α-tubulin antibodies and imaged by confocal microscopy. Scale bar, 20 μm. ( e ) Inhibition of both Gα and Gβ are required to block LPA-induced activation of GEF-H1 exchange activity. RhoA nucleotide exchange rates were measured in lysates from HEK293T cells expressing combinations of GEF-H1–eGFP, Tctex-1, rgRGS domain and βARKct peptide, with or without LPA stimulation, as indicated. The s.d. of at least three independent replicates are shown along with P values from pairwise t -tests. Full size image Gα or Gβ is sufficient to release GEF-H1 from microtubules Having demonstrated that either Gβ or Gα can activate GEF-H1, we queried whether both subunits are required in vivo for stimulation of GEF-H1 by ligand-induced activation of GPCRs. Following stimulation with thrombin, GEF-H1 was immunoprecipitated from lysates of starved HEK293T cells expressing the rgRGS domain (to sequester Gα 12/13 ) [18] , [19] and/or βARKct (to block Gβ) [16] . The resulting immune complexes were probed for endogenous DIC as a marker of GEF-H1 localization to the microtubule-associated dynein–protein complex. While endogenous DIC was co-immunoprecipitated with Flag-GEF-H1 from starved HEK293T cells ( Fig. 5c ), the amount of DIC associated with GEF-H1 was markedly reduced after 5 min treatment with thrombin ( Fig. 5c ). Expression of either rgRGS or βARKct alone had little impact on thrombin’s ability to disrupt the GEF-H1–DIC interaction, however, co-expression of both rgRGS and βARKct blocked the disruptive effect of thrombin on the GEF-H1–DIC complex ( Fig. 5c ). In parallel experiments, we examined the localization of GEF-H1–eGFP following thrombin treatment in cells expressing the rgRGS domain or the βARKct peptide. We observed that neither the rgRGS domain nor the βARKct peptide alone were sufficient to block the relocalization of GEF-H1 by thrombin, however, the expression of both inhibitory proteins had a potent blocking effect on GEF-H1 relocalization ( Fig. 5d ). These results provide evidence that either Gα or Gβ is sufficient to trigger the displacement of GEF-H1 from the microtubules. Finally, we used the rgRGS domain and/or the βARKct peptide to examine whether Gβ and Gα exhibit functionally redundant or cooperative roles in the GPCR-stimulated activation of GEF-H1. The inhibitory effect of Tctex-1 on GEF-H1 exchange activity was relieved by treatment of cells with LPA, and this was not impacted by expression of rgRGS or βARKct alone ( Fig. 5e ). However co-expression of rgRGS and βARKct together blocked the ability of LPA to relieve Tctex-1 inhibition of GEF-H1, further suggesting that either Gα or Gβ is sufficient to induce GEF-H1 activation. GEF-H1 associates with and is dephosphorylated by PP2A A clue as to the identity of the phosphatase that dephosphorylates GEF-H1 Ser885 was obtained from a systematic survey of all PP2A catalytic, scaffolding and regulatory subunit interactions. In this screen, Flag-tagged components of the PP2A holoenzyme were expressed in 293 Flp-In T-REx cells, and used for affinity purification coupled to mass spectrometry. GEF-H1 was detected with several of the bait proteins in this screen ( Supplementary Table I ). Spectral counts were extracted for GEF-H1 and normalized to spectral counts for the PP2A-scaffolding A subunit ( PPP2R1A ) to control for differences in expression of the different regulatory subunits. While GEF-H1 was readily recovered with both the catalytic and the scaffolding subunits, it only co-purified with members of one of the regulatory (B) families, the B′ regulatory subunits PPP2R5A, PPP2R5B and PPP2R5E ( Fig. 6a ), suggesting specificity in the regulatory subunit selection. We validated the interactions between GEF-H1 and the PP2A subunits by co-immunoprecipitation and showed that endogenous GEF-H1 and endogenous PP2A catalytic subunit proteins bind to one another ( Fig. 6b ). Next, we confirmed the specificity in regulatory subunit selection by co-immunoprecipitation followed by immunoblotting using the stable cell lines used in Fig. 6a : Flag-tagged PP2A catalytic subunit and B′ regulatory subunit, but not B, B′′ or B′′′ subunits, each precipitated endogenous GEF-H1 ( Fig. 6c ). To map the regions of GEF-H1 involved in PP2A binding, we expressed truncated variants of GEF-H1 and probed for the catalytic subunit of PP2A in GEF-H1 immune complexes ( Fig. 6d ). The endogenous PP2Ac subunit was present in precipitates of full-length GEF-H1, the Dbl-homology (DH) and pleckstrin-homology (PH) domain (236–572) and the PH domain (473–572), but not in complexes formed by the DH domain alone, thus localizing the PP2Ac-binding site to the PH domain of GEF-H1 ( Fig. 6d ). 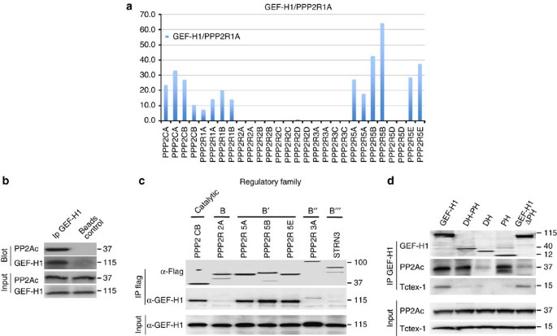Figure 6: The interaction of PP2A with GEF-H1 is inducible. (a) Identification of GEF-H1 as an interaction partner with specific PP2A subunits. Spectral counts from affinity purification and mass spectrometry (AP-MS) experiments for GEF-H1 and the A subunit PPP1R1A using the catalytic (PPP2CA, PPP2CB), scaffolding (PPP2R1A, PPP2R1B) and indicated regulatory B subunits as bait. Baits are represented on thexaxis with two biological replicates performed per bait. Theyaxis indicates GEF-H1 spectra normalized to PPP2R1A (number spectra for GEF-H1/number spectra for PPP2R1A) × 100. Values were plotted independently for each replicate to assess the reproducibility of the measurements. (b) Endogenous GEF-H1 and endogenous catalytic subunit of PP2A interact. Wild-type MEF cells growing in DMEM 10% FBS were lysed and GEF-H1 immune complexes were probed for endogenous PP2A catalytic subunit with anti-PP2Ac antibodies. Total GEF-H1 and PP2Ac expression levels are shown. (c) GEF-H1 interacts with PP2A catalytic and B′ subunits. Flp-In T-RexHEK293 cells, each stably expressing a distinct Flag-PP2A subunit, were lysed and PP2A subunits were immunoprecipitated with anti-Flag antibodies (row 1). PP2A subunit complexes were probed for endogenous GEF-H1 using anti-GEF-H1 antibodies (row 2). (d) PP2A binds to the pleckstrin-homology (PH) domain of GEF-H1. Flag-tagged full-length and truncated variants of GEF-H1 (DH, Dbl-homology; PH, pleckstrin-homology) were precipitated using anti-Flag antibodies (row 1). These complexes were probed for the presence of the endogenous catalytic subunit of PP2A using anti-PP2Ac antibodies (row 2). GEF-H1 and PP2Ac levels in cell lysates are shown (rows 3 and 4). Figure 6: The interaction of PP2A with GEF-H1 is inducible. ( a ) Identification of GEF-H1 as an interaction partner with specific PP2A subunits. Spectral counts from affinity purification and mass spectrometry (AP-MS) experiments for GEF-H1 and the A subunit PPP1R1A using the catalytic (PPP2CA, PPP2CB), scaffolding (PPP2R1A, PPP2R1B) and indicated regulatory B subunits as bait. Baits are represented on the x axis with two biological replicates performed per bait. The y axis indicates GEF-H1 spectra normalized to PPP2R1A (number spectra for GEF-H1/number spectra for PPP2R1A) × 100. Values were plotted independently for each replicate to assess the reproducibility of the measurements. ( b ) Endogenous GEF-H1 and endogenous catalytic subunit of PP2A interact. Wild-type MEF cells growing in DMEM 10% FBS were lysed and GEF-H1 immune complexes were probed for endogenous PP2A catalytic subunit with anti-PP2Ac antibodies. Total GEF-H1 and PP2Ac expression levels are shown. ( c ) GEF-H1 interacts with PP2A catalytic and B′ subunits. Flp-In T-RexHEK293 cells, each stably expressing a distinct Flag-PP2A subunit, were lysed and PP2A subunits were immunoprecipitated with anti-Flag antibodies (row 1). PP2A subunit complexes were probed for endogenous GEF-H1 using anti-GEF-H1 antibodies (row 2). ( d ) PP2A binds to the pleckstrin-homology (PH) domain of GEF-H1. Flag-tagged full-length and truncated variants of GEF-H1 (DH, Dbl-homology; PH, pleckstrin-homology) were precipitated using anti-Flag antibodies (row 1). These complexes were probed for the presence of the endogenous catalytic subunit of PP2A using anti-PP2Ac antibodies (row 2). GEF-H1 and PP2Ac levels in cell lysates are shown (rows 3 and 4). Full size image We sought to determine whether PP2A was the phosphatase responsible for the dephosphorylation required for GEF-H1 activation. Flag-GEF-H1 derived from starved HEK293T cells was highly phosphorylated, as determined by an antibody recognizing the phosphorylated 14-3-3-binding motif ( Fig. 7a ). Immunopurified Flag-GEF-H1 was then incubated with 0.1 U of recombinant PP2A catalytic subunit or buffer control, and a time course of the phosphorylation state was followed by western blot using phospho 14-3-3-binding motif recognition antibody. Dephosphorylation of GEF-H1 at the 14-3-3 consensus sites by recombinant PP2Ac occurred within 10 min ( Fig. 7a ), demonstrating that GEF-H1 can serve as a PP2A substrate. Together, these data demonstrate that GEF-H1 physically interacts with PP2A, which can dephosphorylate 14-3-3-binding sites in vitro . Since the inhibited state of GEF-H1 is associated with phosphorylation of the driver 14-3-3 site Ser885, and mutation of this site (Ser885A) causes constitutive activation of GEF-H1 (ref. 6 ), we wanted to determine whether thrombin treatment specifically induced dephosphorylation of Ser885. Starved cells were treated with thrombin and cells were lysed over a time course of 45 min, and immunoblotted with a phospho-Ser885-specific GEF-H1 antibody. Ser885 phosphorylation was detected in starved cells, but decreased after 5 min of thrombin treatment ( Fig. 7b ). GEF-H1 dephosphorylation at Ser885 was transient, with the return of phosphorylation by 10 min, suggesting that GEF-H1 is active for only a brief period of time. 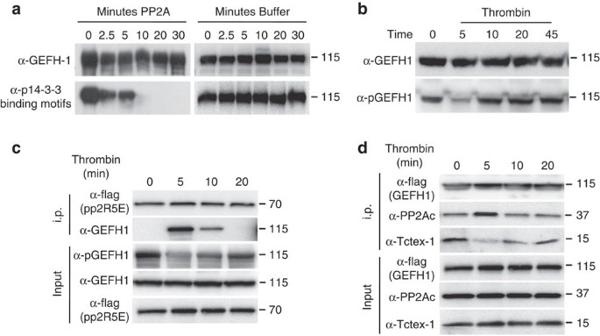Figure 7: PP2A dephosphorylates GEF-H1 at 14-3-3-binding sites in response to thrombin. (a) PP2A dephosphorylates GEF-H1in vitro. Cells expressing Flag-GEF-H1 were treated with calyculin, GEF-H1 immune complexes were immunoprecipitated and incubated with recombinant catalytic subunit of PP2A for different time periods. GEF-H1 immunocomplexes were probed for GEF-H1 and for phosphorylated 14-3-3-binding motifs using anti-Flag or anti-phospho14-3-3 recognition site antibodies, respectively. (b) Thrombin treatment induces rapid but transient dephosphorylation of GEF-H1 at Ser885. Cells were treated with thrombin and lysates probed with an anti-GEF-H1 phosphoSer885 antibody. (c,d) Thrombin treatment induces association between PP2A and GEF-H1. (c) Cells stably expressing Flag-PPP2R5E were treated with thrombin for different times. Flag-PPP2R5E immune complexes were probed for the presence of endogenous GEF-H1. Lysates were probed for total levels of Flag-PPP2R5E, GEF-H1 and phosphoS885. (d) Cells expressing Flag-GEF-H1 were treated with thrombin for different times. Flag-GEF-H1 immune complexes were isolated and probed for the presence of the endogenous catalytic subunit of PP2A and for endogenous Tctex-1. Lysates were probed for total levels of Flag-GEF-H1, PP2Ac and Tctex-1. Figure 7: PP2A dephosphorylates GEF-H1 at 14-3-3-binding sites in response to thrombin. ( a ) PP2A dephosphorylates GEF-H1 in vitro . Cells expressing Flag-GEF-H1 were treated with calyculin, GEF-H1 immune complexes were immunoprecipitated and incubated with recombinant catalytic subunit of PP2A for different time periods. GEF-H1 immunocomplexes were probed for GEF-H1 and for phosphorylated 14-3-3-binding motifs using anti-Flag or anti-phospho14-3-3 recognition site antibodies, respectively. ( b ) Thrombin treatment induces rapid but transient dephosphorylation of GEF-H1 at Ser885. Cells were treated with thrombin and lysates probed with an anti-GEF-H1 phosphoSer885 antibody. ( c , d ) Thrombin treatment induces association between PP2A and GEF-H1. ( c ) Cells stably expressing Flag-PPP2R5E were treated with thrombin for different times. Flag-PPP2R5E immune complexes were probed for the presence of endogenous GEF-H1. Lysates were probed for total levels of Flag-PPP2R5E, GEF-H1 and phosphoS885. ( d ) Cells expressing Flag-GEF-H1 were treated with thrombin for different times. Flag-GEF-H1 immune complexes were isolated and probed for the presence of the endogenous catalytic subunit of PP2A and for endogenous Tctex-1. Lysates were probed for total levels of Flag-GEF-H1, PP2Ac and Tctex-1. Full size image We then examined whether the interaction between PP2A subunits and GEF-H1 increased in response to thrombin treatment, and whether the kinetics of the interaction correlated with the transient dephosphorylation of Ser885. Starved HEK293T cells expressing Flag-tagged PPP2R5E B′ subunit were treated with thrombin and lysed at different time points. Flag-PPP2R5E B′ immunoprecipitates were probed for endogenous GEF-H1. We observed a switch-like induction of GEF-H1 association with the B′ subunit at 5 min following thrombin treatment ( Fig. 7c ). This interaction was reduced at 10 min and was undetectable after 20 min of thrombin treatment ( Fig. 7c ). The GEF-H1:PP2A interaction was anti-correlated with Ser885 phosphorylation ( Fig. 7c , third panel), with the protein complex assembling to its maximum at 5 min following thrombin treatment and decreasing towards baseline thereafter. We observed similar kinetics in the interaction between GEF-H1 and the endogenous PP2A catalytic subunit following thrombin treatment ( Fig. 7d ). Importantly, the levels of GEF-H1 associated with the microtubule dynein complex, as measured by the association of GEF-H1 with Tctex-1, decreased in response to thrombin ( Fig. 7d ). These results show that PP2A and GEF-H1 form a dynamic complex in response to thrombin, which is temporally correlated to dephosphorylation of the GEF-H1 negative regulatory site Ser885, loss of dynein interaction and redistribution from the microtubule array. Microtubule depolymerization-independent GEF-H1 activation Our results suggest a model where GEF-H1 activation results from disruption of the GEF-H1:dynein complex by G-protein subunits in the absence of microtubule depolymerization [6] , [7] . To test this model, we next determined whether Taxol-induced stabilization of microtubules could inhibit LPA or thrombin-mediated activation of GEF-H1. We measured the effect of Taxol on GPCR-mediated GEF-H1 dephosphorylation, stress fibre formation and GEF activation. Starved HEK293T cells were pre-treated with Taxol and then stimulated with thrombin. Lysates were recovered at different time intervals and probed for the levels of GEF-H1 pSer885. We found that Taxol did not affect the kinetics or the magnitude of thrombin-induced GEF-H1 dephosphorylation compared with untreated control cells ( Fig. 8a ). Similarly, we examined whether Taxol could suppress LPA or thrombin-induced GEF-H1 redistribution from the microtubule array and stress fibre formation. GEF-H1 knockout MEFs were transfected with GEF-H1–eGFP, starved for 3 days, exposed to Taxol and visualized by confocal microscopy after LPA or thrombin treatment. Pretreatment of cells with Taxol failed to suppress LPA or thrombin-stimulated GEF-H1 redistribution from the microtubule to the cytoplasm and the formation of stress fibres ( Fig. 8b,d ). To ensure that the microtubules were not undergoing rapid cycles of depolymerization/repolymerization, even in the presence of Taxol, we expressed GEF-H1–eGFP together with cherry tubulin, treated the cells with Taxol and visualized them by real-time confocal microscopy. GEF-H1 rapidly relocalized into a cytoplasmic vesicular pattern within 60 s of LPA stimulation, in the absence of microtubule depolymerization ( Fig. 8c ). Moreover, the microtubule stabilizing effect of Taxol could not antagonize activation of GEF-H1 by LPA or thrombin ( Fig. 8e ; Supplementary Fig. 5 ). These data provide evidence that GPCR-mediated activation of GEF-H1 does not require disassembly of the microtubule array. Since the microtubule-depolymerizing agent nocodazole activates GEF-H1 by direct microtubule depolarization ( Fig. 8b , third row and Fig. 8e ), we investigated whether pretreatment of cells with Taxol could suppress this effect. We observed that pretreatment with Taxol prior to exposure to nocodazole blocked the ability of nocodazole to stimulate both stress fibre formation ( Fig. 8b ) and GEF-H1 activation ( Fig. 8e ). 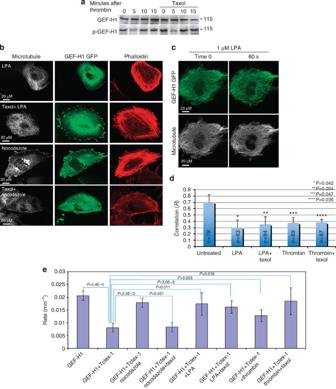Figure 8: GPCR-mediated activation of GEF-H1 does not require microtubule depolymerization. (a) Thrombin-induced GEF-H1 dephosphorylation is independent of microtubule depolymerization. Cells were treated with thrombin for different times with or without Taxol pretreatment. Lysates were probed for GEF-H1 and phosphoSer885 GEF-H1 levels by western blot. (b) Taxol suppresses nocodazole but not LPA-stimulated redistribution of GEF-H1 from the microtubule to the cytoplasm. GEF-H1−/−MEFs were transfected with GEF-H1–eGFP, starved for 3 days and then treated with LPA, thrombin or nocodazole with or without 24-h Taxol pretreatment. Cells were fixed and stained with anti-phalloidin and anti-tubulin antibodies and imaged by confocal microscopy. Scale bar, 20 μm. (c) LPA-induced GEF-H1 relocalization is independent of microtubule depolymerization. Real-time live-cell images of GEF-H1 and microtubules following LPA stimulation. GEF-H1−/−MEFs were transiently transfected with GEF-H1–eGFP and Cherry tubulin, treated by Taxol then stimulated with LPA. Scale bar, 20 μm. (d) The correlation coefficient (R) measuring co-localization between GFP (GEF-H1) and polymerized microtubules inbwas determined in at least 63 cells from three independent experiments. Error bars represent s.d. of at least three independent replicates, andPvalues derived from pairwiset-tests are indicated. (e) Taxol suppresses nocodazole—but not LPA—or thrombin-induced activation of GEF-H1 exchange activity. RhoA nucleotide exchange rates were measured in the lysates derived from HEK293T cells overexpressing GEF-H1–eGFP or co-expressing GEF-H1–eGFP and Flag-Tctex-1, untreated or treated with LPA, thrombin or 20 μM nocodazole, with or without 24-h pretreatment with Taxol. The s.d. derived from at least three independent replicates are indicated, withPvalues from pairwiset-tests. Figure 8: GPCR-mediated activation of GEF-H1 does not require microtubule depolymerization. ( a ) Thrombin-induced GEF-H1 dephosphorylation is independent of microtubule depolymerization. Cells were treated with thrombin for different times with or without Taxol pretreatment. Lysates were probed for GEF-H1 and phosphoSer885 GEF-H1 levels by western blot. ( b ) Taxol suppresses nocodazole but not LPA-stimulated redistribution of GEF-H1 from the microtubule to the cytoplasm. GEF-H1 −/− MEFs were transfected with GEF-H1–eGFP, starved for 3 days and then treated with LPA, thrombin or nocodazole with or without 24-h Taxol pretreatment. Cells were fixed and stained with anti-phalloidin and anti-tubulin antibodies and imaged by confocal microscopy. Scale bar, 20 μm. ( c ) LPA-induced GEF-H1 relocalization is independent of microtubule depolymerization. Real-time live-cell images of GEF-H1 and microtubules following LPA stimulation. GEF-H1 −/− MEFs were transiently transfected with GEF-H1–eGFP and Cherry tubulin, treated by Taxol then stimulated with LPA. Scale bar, 20 μm. ( d ) The correlation coefficient ( R ) measuring co-localization between GFP (GEF-H1) and polymerized microtubules in b was determined in at least 63 cells from three independent experiments. Error bars represent s.d. of at least three independent replicates, and P values derived from pairwise t -tests are indicated. ( e ) Taxol suppresses nocodazole—but not LPA—or thrombin-induced activation of GEF-H1 exchange activity. RhoA nucleotide exchange rates were measured in the lysates derived from HEK293T cells overexpressing GEF-H1–eGFP or co-expressing GEF-H1–eGFP and Flag-Tctex-1, untreated or treated with LPA, thrombin or 20 μM nocodazole, with or without 24-h pretreatment with Taxol. The s.d. derived from at least three independent replicates are indicated, with P values from pairwise t -tests. Full size image We report here a multistep mechanism for GPCR-mediated activation of the RhoGEF GEF-H1. We show that both Gα and Gβγ subunits operate in a concerted manner to activate GEF-H1 through its displacement from the microtubule array, where it is anchored in an inhibited state by the dynein motor light-chain Tctex-1. In addition, we have discovered that following thrombin stimulation, the PP2A phosphatase associates with GEF-H1 and dephosphorylates the negative regulatory 14-3-3-binding site, Ser885. RhoGEFs are activated by G-protein subunits through a variety of different mechanisms [13] . For example, Gα 12/13 subunits activate p115-RhoGEF, LARG and PDZ-RhoGEF [18] , Gαq/11 activates p63RhoGEF and TrioC, whereas Gβγ can directly bind and activate P-Rex1 and P-Rex2, p114RhoGEF and Arhgef5 (refs 13 , 22 ). Gα 12/13 subunits bind to their target proteins through a conserved domain called the RGS. There are over 39 mammalian RGS- and RH-domain-containing proteins ranging from small proteins comprised solely of an RGS domain to multi-domain proteins, which serve as scaffolds to diversify downstream signalling events. The canonical RGS domain consists of a nine-α-helix bundle, which in some instances can stabilize the Gα 12/13 transition state required to accelerate the hydrolysis of GTP, which inactivates Gα thus controlling the longevity of G-protein signalling [23] , [24] , [25] , [26] . The RhoGEFs p115-RhoGEF, LARG and PDZ-RhoGEF bind to Gα 12/13 subunits through a RH domain [27] contained in their peptide sequence. The RH domains of the p115RhoGEF [28] and the PDZ-RhoGEF [29] share a conserved core with the RGS domain, but possess additional N- and C-terminal extensions that mediate a distinct mode of interaction with Gα. Gα 12/13 localizes GEFs to the plasma membrane or stimulates GEF activity directly through the release of an autoinhibitory domain or both [18] , [30] , [31] , [32] , [33] . GEF-H1 lacks a canonical RGS domain, nevertheless, in this study, we have shown that active Gα 12/13 binds to a region encompassing the first 240 amino acids of GEF-H1 and stimulates its intrinsic exchange activity. We carefully examined whether this region of GEF-H1 shares any structural features of a RH domain, however, the N terminus of GEF-H1 cannot be aligned with RH-containing sequences present in PDZ-RhoGEF and p115-RhoGEF. Furthermore, the DISOPRED algorithm [34] predicts that this region is intrinsically disordered except for residues 40–85, which comprise a conserved C1 domain predicted to form a zinc-finger-like structure. Furthermore, GEF-H1 lacks the IIG and EDF/YD/E motifs that typify the RH domains present in other RhoGEFs. Our pull-down data ( Fig. 4a,b ) indicated that residues 1–87 (which include the C1 domain) bind Gα weakly, whereas residues 87–985 bind Gα almost as well as 1–985. These results strongly argue that Gα binding to GEF-H1 involves an intrinsically disordered region in the N-terminal portion of GEF-H1, which may undergo binding-coupled folding. Such protein–protein interactions involving intrinsically disordered regions have been seen in many signalling proteins and transcription factors [35] . More comprehensive understanding of this unique mode of Gα interaction awaits further structural studies to elucidate the detailed binding interface of GEF-H1 and Gα 12/13 . We have demonstrated that the consequences of Gα binding to GEF-H1 include displacement of GEF-H1 from the microtubule array. This effect is most likely a direct result of competitive binding between Gα 12/13 and Tctex-1, since they share an overlapping binding site within the N terminus of GEF-H1. Gα 12/13 activates GEF-H1 first by displacing GEF-H1 from the microtubule-associated inhibited sink, however, it is possible that Gα 12/13 binding to the N terminus of GEF-H1 might also relieve a potential negative regulatory mechanism in a manner similar to the regulation of the RH-family of GEFs. In addition to the action of Gα, we have shown Gβγ subunits activate GEF-H1 by targeting the Tctex-1:DIC-binding interface. Tctex-1 was found to bind to Gβγ subunits in a functional genetic screen looking for receptor-independent activators of G-proteins called activator of G-protein signalling [14] . In a subsequent study, Sachdev et al . [15] found that Gβγ binds to a dynein-free cytoplasmic fraction of Tctex-1. They showed that Gβ competes with the DIC to displace Tctex-1 from the dynein motor complex. Our data demonstrate that Gβγ subunits operating downstream of thrombin or LPA receptors dispace and activate GEF-H1 through a similar mechanism. We propose that free Gβγ subunits bind to Tctex-1, resulting in the displacement of Tctex-1 and GEF-H1 from DIC and the dynein complex. Therefore, both Gα and Gβγ collaborate to disrupt the GEF-H1:Tctex-1:DIC inhibited complex by competing with the GEF-H1:Tctex-1 and Tctex-1:DIC interfaces, respectively. To our knowledge, this is the first report of a system in which both the Gα and Gβ subunits signal to activate a pathway by engaging distinct components of the same complex. Nocodozole-induced microtubule depolymerization potently activates GEF-H1 (refs 5 , 6 , 7 ), thus GEF-H1 activity during mitosis may be a consequence of the change in microtubule dynamics during the reorganization of stable interphase microtubules into the mitotic spindle [36] . Our data demonstrate that GEF-H1 can be activated in interphase through a second mechanism that is independent of microtubule disassembly. We show that LPA or thrombin treatment leads to the acute relocalization of GEF-H1 off the microtubule array without evidence of microtubule disruption. Whereas Taxol suppressed the effects of nocodazole-mediated microtubule depolymerization and GEF-H1 activation, it had no effect on inhibiting LPA- or thrombin-mediated microtubule relocalization or activation of GEF-H1. Therefore, disruption of the GEF-H1:Tctex-1-inhibited complex following LPA treatment by the concerted actions of Gα and Gβγ are sufficient to activate GEF-H1 in the absence of microtubule depolymerization. A similar phenomenon has recently been reported where the activation of GEF-H1 following the application of tensional force on cells was independent of microtubule depolymerization [10] . Thrombin-induced partial depolymerization of microtubules has been described in endothelial cells [2] . We observed such partial depolymerization of microtubules in response to thrombin treatment only at time points after GEF-H1 had already been released from the microtubules. Moreover, blocking this depolymerization by Taxol did not prevent GEF-H1 relocalization. Interestingly, GEF-H1 displacement from microtubules may contribute to microtubule depolymerization in response to thrombin, as GEF-H1 has been reported to promote microtubule stability [37] . GEF-H1’s activity in normal cells is tightly regulated through phosphorylation [3] , [7] , [21] , [38] . In a previous publication, we found that PKA phosphorylates and inhibits GEF-H1 by creating a 14-3-3-binding site [3] , which strongly suggests that a cellular phosphatase(s) is involved in the activation of GEF-H1. In this study, we provide evidence that the PP2A phosphatase positively regulates GEF-H1 by dephosphorylating Ser885. We show that GEF-H1 associates with the catalytic (C), scaffold (A) and B′ regulatory subunits of the PP2A heterotrimer in cells, and that the recombinant PP2A catalytic subunit was competent to dephosphorylate the 14-3-3-binding site on GEF-H1 in vitro . Moreover, we demonstrated that activation of cells with either thrombin or LPA induced a transient GEF-H1:PP2A interaction that was temporally correlated with both dephosphorylation of Ser885 and stress fibre formation. The precise mechanisms by which G-protein subunits trigger the assembly of GEF-H1 with PP2A remain to be established. In summary, we describe a novel multistep process by which the RhoGEF GEF-H1 is activated downstream of GPCR stimulation. We show that G-protein subunits engage in the disassembly of the GEF-H1:Tctex-1:DIC complex, which tethers GEF-H1 locked in an inhibited state to polymerized microtubules. The displacement of GEF-H1 from the microtubule array corresponds with its assembly with PP2A phosphatase subunits required for the dephosphorylation of a negative regulatory 14-3-3-binding site in the carboxyterminus of GEF-H1. We conjecture that the multiple molecular events required for GEF-H1 activation has evolved as a mechanism to ensure a highly restricted temporal and spatial activation of the Rho pathway downstream of GPCR ligand stimulation. Expression constructs Full-length GEF-H1 (accession no. AF177032) or truncated versions (as described in the figures) were cloned into the pFlag-CMV2 vector (Sigma). Complementary DNAs for all full-length and truncated versions of GEF-H1 and Δ87-151GEF-H1 were cloned into pcDNA3.1-His/Myc vector (Invitrogen). eGFP-tagged GEF-H1 and Tctex-1 were constructed by cloning full-length GEF-H1 or Tctex-1 (accession no. NM_174620) into peGFP-C1 (Invitrogen). GEF-H1, Δ151GEF-H1 and Tctex-1 were cloned into the BglII/AgeI and BglII/EagI sites of pCMV-HA-VC155 and pCMV-HAVN173, respectively. Cell culture and transfection MEFs derived from GEF-H1 −/− (ref. 6 ) or wild-type littermate embryos and HEK293T cells were cultured in Dulbecco's modified Eagle's medium (DMEM, Life Technologies Inc.) supplemented with 10% fetal bovine serum (FBS) (HyClone). MEFs and Rat2 cells were transfected using Effectene (QIAGEN), and HEK293T using Polyfect, according to the manufacturer's instructions. All cultures were maintained in a 5% CO 2 environment at 37 °C. For cell spreading and attachment analyses, cells were propagated at low passage number in the presence of DMEM with 10% FBS. Antibodies Rabbit anti-DYNLT1 antibody (anti-Tctex-1) was purchased from Proteintec (11954-1-ap). Polyclonal sheep anti-GEF-H1 antibodies were described previously [36] . Mouse anti-vinculin antibody (anti-vinculin) was purchased from Sigma (V9131), anti-14-3-3 from Santa Cruz (sc-1657), anti-PP2A catalytic alpha from Becton Dickinson (05–421) and anti-phospho-Ser 14-3-3-binding motif from Cell Signaling Technology (4E2, 9606). Rabbit anti-phospho-S885 antibody was from Cell Signaling Technology. Mouse monoclonal antibody directed against bovine α-tubulin (236-10501, A-11126), Pacific Blue anti-mouse IgG (P31582), Texas Red anti-rabbit IgG (T-2767), Texas Red anti-mouse IgG (T-862), Texas Red phalloidin (T7471), Alexa Fluor 350 phalloidin (A22281) and Alexa Fluor 594 donkey anti-sheep IgG (A-11016) were obtained from Invitrogen. Western blotting and immunofluorescence was performed using the following primary antibodies; anti-Flag (M2, F3165, Sigma), anti-His (H15, sc-803), anti-GST (B-14, sc-138), anti-Myc (Sigma, M4439), anti-PP2Ac (Millipore, 05–421) and anti-HA (H6908, Sigma). HRP-conjugated anti-mouse or anti-rabbit secondary antibodies were from GE Healthcare. Supplementary Figs 7–12 show full scans of the western blots presented in the main figures. Immunofluorescence imaging Cells grown on glass coverslips were treated as indicated in the corresponding figure legends and fixed with 4% paraformaldehyde for 10 min, washed three times with phosphate-buffered saline (PBS) and permeabilized with 0.1% Triton-X-100 for 5 min. The coverslips were blocked with 0.5% w/v bovine serum albumin (BSA) in PBS for 1 h at room temperature and incubated with primary antibody (anti-DYNLT1 1:400, sheep anti-GEF-H1 1:150, anti-tubulin 1:300 and anti-vinculin 1:400) or Texas Red phalloidin (1:400) in 0.5% BSA/PBS at 37 °C for 30 min or at 4 °C overnight. Coverslips were washed three times with PBS and incubated with secondary antibody (1:500) at 37 °C for 1 h. For double labelling, slides were stained sequentially with primary and secondary antibodies at 37 °C for 30 min, followed by 4',6-diamidino-2-phenylindole (Molecular Probes, Invitrogen) to stain nuclei. Slides were mounted using GelTol mounting medium (Shandon Immunon, Thermo Electron Corporation). Confocal imaging was performed with an Olympus IX81 inverted microscope using a × 60 zoom × 3(1.4 NA; PlanApo, Nikon) objective, and FluoView software (Olympus, Tokyo, Japan). Resolution was 512 × 512 with 12 bits per pixel. Excitation wavelengths used for GFP, Texas Red, 4',6-diamidino-2-phenylindole or Pacific Blue were 473, 559, 358 and 405 nm, respectively. All images in each set of experiments were acquired with the same microscope sensitivity settings. All images compared within each figure panel were acquired on the same day, with identical staining conditions, gain and contrast setting, and same magnification (except Fig. 1c ). All statistical analyses were derived from 60 or more images from three independent experiments for each treatment condition. NMR-based GEF assay To measure GEF activity in lysates of mammalian cells, real-time NMR GEF assays were performed [6] , [17] . Nucleotide exchange assays were carried out at 20 °C with 0.4 mM 15 N-labelled RhoA (residues 1–181) in NMR buffer (20 mM HEPES, 100 mM NaCl, 5 mM MgCl 2 , 2 mM Tris (2-carboxyethyl) phosphine, 10% D 2 O, pH 7.0) using a Bruker 600 MHz NMR spectrometer equipped with a 1.7-mm microcryoprobe. Successive 1 H- 15 N-HSQC spectra (4 scans, 10 min per spectrum) were collected and seven pairs of guanosine diphosphate (GDP)/GTPγS-specific peaks (V9, Q29, A56, S73, D87, T163 and W158) were used to determine the fraction of GDP-bound RhoA in each spectrum ( Supplementary Fig. 6 ). Data were fitted to a single-phase exponential decay function to obtain the exchange rate. HEK293T cells were transfected with the indicated constructs for 48 h, and the GEF activity in lysates was measured by harvesting cells in a minimal volume (for example, 150 μl for a 6-cm plate) of lysis buffer (1% Triton-X, 10% glycerol, 50 mM HEPES pH 7.5, and Complete Protease Inhibitor cocktail (Roche)) to achieve high total protein concentration (~10 μg μl −1 ). All cell lysates were freshly prepared immediately before performing assays, and partially clarified by centrifugation (16,000 g , 30 s). The amount of GEF-H1 in each assay was standardized by eGFP fluorescence of the lysate measured by a Shimadzu RF-5301PC spectrofluorophotometer. To compare endogenous cellular GEF activity, total cellular protein in lysates was standardized using the Bradford assay. To initiate nucleotide exchange, 2 mM GTPγS and lysate were added to 15 N RhoA-GDP. Intrinsic RhoA nucleotide exchange was measured by adding lysis buffer. Where indicated, HEK293 cells were treated prior to harvesting as follows: nocodazole (20 μM, 10 min), Taxol (10 μM), LPA (1 μM, 30 min) and thrombin (3 U ml −1 , 1 h). Image analysis Image analysis for co-localization was performed with the cell profiler v2.0 1 using the ‘MeasureCorrelation’ module for correlation. Focal adhesion counts were performed using ImageJ v1.4q 2 ( http://rsb.info.nih.gov/ij/index.html ). Vinculin-stained cell images were transformed to 16 bits and the background was subtracted using the ‘background subtractor’ plugin 3. Then they were transformed into binary images and focal adhesions were identified using the find maxima tool (Noise tolerance of 20). Paired Student’s t -tests (ref. 39 ) were performed to determine statistical significance between samples. Experiments were performed at least three times, and means with P <0.05 were considered statistically significant. The correlation coefficient ( R ) measuring co-localization was determined from three independent experiments. Error bars represent s.d. of at least three independent replicates, and P values derived from pairwise t -tests are indicated. Full-length GEF-H1 expression and purification protocol Full-length GEF-H1 with a His 6 tag and an N -terminal immunoglobulin-binding protein (BiP) secretion signal sequence was expressed in Drosophila S2 cells using the pMTTEVA vector [6] . S2 cells were cultured in serum-free media and induced with 6 μM CdCl 2 at a density of 5 × 10 6 cells per ml for 4 days. GEF-H1 was captured with Ni 2+ -NTA resin and further purified by anion-exchange (HiTrap Q) and size-exclusion chromatography (Superdex 200). Purified recombinant Gα 13 was a kind gift from P. Sternweis (UT Southwestern Medical Center). Cell treatments Cells were starved for 5 days in the absence of serum and treated in DMEM containing 20 mM HEPES and 0.5 mg ml −1 fatty acid-free BSA (A8806, Sigma). LPA obtained from Sigma (7260) was suspended in Hank’s buffered saline solution containing 0.5 mg ml −1 fatty acid-free BSA and 20 mM HEPES to a stock concentration of 1 mM. Cells were treated with 1 μM LPA for 30 min or as indicated in the figures. Bovine thrombin (605157) was purchased from Calbiochem and reconstituted to a concentration of 1 U μl −1 . Cells were treated with 3 U ml −1 thrombin for 1 h or as indicated in the figures. Proteomics analyses Flp-In T-Rex 293 cells (Invitrogen) were stably transfected with N-terminally-FLAG-tagged PP2A constructs and protein expression was induced by tetracycline addition. FLAG-tagged proteins and their putative interaction partners were recovered by immunoprecipitation on anti-FLAG magnetic beads [40] . Mass spectroscopy Samples digested on beads were acidified and loaded onto home-packed C18 capillary columns (75 μm inner diameter). HPLC columns were placed in-line in front of an LTQ mass spectrometer (Thermo) equipped with a Nanosource (Proxeon) for data-dependent acquisition over a 2-h acetonitrile 2–40% gradient [41] . Acquired RAW files were converted to mgf format using ProteoWizard [42] , and searched with the Mascot search engine (Matrix Science, London, UK, version 2.3.02) against the human RefSeq database supplemented with the RefSeq adenovirus entries (release 45) with a precursor ion mass tolerance of 3.0 and a fragment ion mass tolerance of 0.6. Methionine oxidation and asparagine deamidation were allowed as variable modifications, and trypsin specificity (with one missed cleavage allowed) was selected. The data were analysed in the ‘Analyst’ module of ProHits [43] and exported into Excel files for spectral normalization and manual extraction of the data corresponding to GEF-H1 and PPP2R1A (the remainder of the data set will be the topic of a separate publication). Two biological replicates analyses were performed on each of the baits. Fourteen negative control runs were also performed that consisted of cells expressing the FLAG tag fused to a green fluorescent protein. Importantly, GEF-H1 was not identified in any of the negative control runs. Phosphatase assays For dephosphorylation of GEF-H1 immunoprecipitates with PP2A, cells were lysed in phosphatase lysis buffer (50 mM Tris pH 7.5, 150 mM NaCl, 1 mM EDTA pH 8, 1% v/v NP40, 1 mM dithiothreitol, 1 mM phenylsulfonylfluoride with Complete Protease Inhibitor cocktail (Roche)), and immunoprecipitates were washed twice with lysis buffer then three times with PP2A phosphatase buffer (20 mM HEPES pH 8, 1 mM dithiothreitol and 1 mM MnCl 2 ). Beads were preheated with 100 μl PP2A phosphatase buffer for 10 min at 30 °C prior to the addition of 0.1 U PP2A (Upstate, 14-111) and incubation at 30 °C. Reactions were stopped by washing beads with lysis buffer containing phosphatase inhibitors and boiling beads for 10 min in 2 × sample buffer prior to SDS–polyacrylamide gel electrophoresis. Statistical analyses Values are expressed as means±s.d. Paired Student’s t -tests [39] were performed to determine statistical significance between samples. Experiments were performed at least three times and means with P <0.05 were considered statistically significant. How to cite this article: Meiri, D. et al . Mechanistic insight into GPCR-mediated activation of the microtubule-associated RhoA exchange factor GEF-H1. Nat. Commun. 5:4857 doi: 10.1038/ncomms5857 (2014).